Probing single- to multi-cell level charge transport inGeobacter sulfurreducensDL-1 Microbial fuel cells, in which living microorganisms convert chemical energy into electricity, represent a potentially sustainable energy technology for the future. Here we report the single-bacterium level current measurements of Geobacter sulfurreducens DL-1 to elucidate the fundamental limits and factors determining maximum power output from a microbial fuel cell. Quantized stepwise current outputs of 92(±33) and 196(±20) fA are generated from microelectrode arrays confined in isolated wells. Simultaneous cell imaging/tracking and current recording reveals that the current steps are directly correlated with the contact of one or two cells with the electrodes. This work establishes the amount of current generated by an individual Geobacter cell in the absence of a biofilm and highlights the potential upper limit of microbial fuel cell performance for Geobacter in thin biofilms. Microbial fuel cells (MFCs) are one of the most progressive alternative energy technologies for the future [1] , [2] , [3] , [4] , [5] , [6] , [7] . The fundamental design behind MFCs has led to systems that can generate hydrogen [8] or electricity directly from aquatic sediments [9] . Electrochemically active bacteria (EAB), such as Shewanella and Geobacter , can transfer electrons from oxidative metabolism of organic sources to electrodes through reduced outer membrane proteins or soluble redox mediators [2] , [10] , [11] , [12] . Although considerable progress has been made in improving MFC performance through the optimization of microbe selection [13] , [14] and fuel cell design [7] , [15] , the complex nature of biofilms in working MFCs has hindered a detailed understanding of charge transport at microbe/electrode and microbe/microbe interfaces [16] , [17] , [18] , [19] . Electron transfer from an EAB to an insoluble electron acceptor (that is, electrode) can occur by either direct (cellular contact with surface or biofilm), mediated (soluble redox compounds such as flavins and/or quinones) or a combination of both mechanisms (secreted mediators in biofilms) [20] . Unlike the mediated electron transfer that occurs when studying Shewanella oneidensis MR-1 (ref. 21 ), Geobacter sulfurreducens has only been associated with direct electron transfer mechanisms either through extracellular pilin decorated with cytochromes or the cell body itself [22] , [23] . Several groups [16] , [18] have actively been debating the mechanism of electron transfer by Geobacter after the publication of data suggesting that protein-based pilin had metal-like conductivity [24] and this metal-like conduction was due to secondary π-stacking of amino acids comprising the pilin itself [25] . Most conductivity and gene expression experiments with Geobacter sp. are based on the formation of biofilms, which has led to a focus on conductivity of the exopolysaccharide matrix more than the amount of current generated from a single cell [26] , [27] . Micro-/nanoelectrode arrays have been demonstrated as a powerful tool for capacitance-based single-bacterium detection/measurement [28] , [29] , and were recently explored as anodes in MFCs to probe extracellular electron transfer in Shewanella species on a single-cell basis [30] , [31] . Our previous work was one of the first measurements of current output from a single bacterium using fabricated nanoelectrodes [30] . These nanostructured electrodes were designed to physically control the contact between a single bacterial cell and the metal electrode surface. However, the soluble mediators present in S. oneidensis cultures obstructed the quantitative characterization of the current output from individual microbes. To address these fundamental issues and to elucidate the intrinsic limits determining power extraction from Geobacter , here we report the first single-cell level electrochemical studies of G. sulfurreducens DL-1 using nanostructured electrodes. Quantized current outputs of 92(±33) and 196(±20) fA were generated from microelectrode arrays confined in isolated wells from the interaction of G. sulfurreducens DL-1 directly with the nanoelectrodes. This work establishes the amount of current generated by an individual Geobacter cell in the absence of a biofilm and highlights the potential upper limit of MFC performance for Geobacter in biofilms. Experimental design and device characterization A new platform has been designed, developed and applied to probe single to multicellular charge transport from a model bacterial system known for extracellular electron transport, G. sulfurreducens DL-1. This bacterium does not release soluble redox mediators [2] and thus is a suitable candidate for single-cell electrochemical studies. An overview of the experimental approach ( Fig. 1a ) illustrates the optically transparent microelectrode arrays confined in separated wells, which allows localized current recordings from multiple electrodes with a controlled microenvironment. The chip fabrication was completed with a two-step photolithography process defining the array of transparent Ti/Au finger electrodes and SU-8 wells sequentially (see Methods). Tilted field-emission scanning electron microscopy image highlights a 100 × 100-μm 2 well containing two parallel finger electrodes with 20 μm interspacing ( Fig. 1b ). The height of SU-8 wall, ~40 μm, is larger than the biofilm thickness that can be formed during our measurement period, thus allowing only the cells confined within the well to be able to make substantial contribution to the local current generation. The exposed area for all electrodes from different wells was designed to be identical and was confirmed by cyclic voltammetry of a ferricyanide solution, which showed comparable steady state currents of ~1 nA ( Fig. 1c ). In contrast, the current recorded from a fully passivated control electrode is <0.1%, indicating minimal leakage from SU-8 layer ( Fig. 1c ). 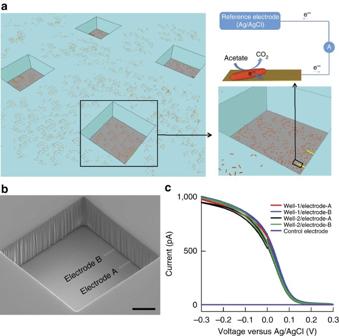Figure 1: Design and characterization of nanoelectrode chip. (a) Schematic of experimental design. (b) Tilted-view scanning electron microscopy image of a 100 × 100 μm2well containing two finger electrodes (electrode A and B) with 20 μm interspacing. The exposed area for each electrode is 24 μm2, and thickness of the SU-8 wall is 40 μm. Scale bar, 20 μm. (c) Cyclic voltammetry measurement of four finger electrodes from two separated wells. From well 1, electrode A (red) and B (blue) and from well 2, electrode A (black) and B (green), and full SU-8 passivation (purple) in 1 mM ferricyanide solution. Figure 1: Design and characterization of nanoelectrode chip. ( a ) Schematic of experimental design. ( b ) Tilted-view scanning electron microscopy image of a 100 × 100 μm 2 well containing two finger electrodes (electrode A and B) with 20 μm interspacing. The exposed area for each electrode is 24 μm 2 , and thickness of the SU-8 wall is 40 μm. Scale bar, 20 μm. ( c ) Cyclic voltammetry measurement of four finger electrodes from two separated wells. From well 1, electrode A (red) and B (blue) and from well 2, electrode A (black) and B (green), and full SU-8 passivation (purple) in 1 mM ferricyanide solution. Full size image Investigation of single-cell current output The G. sulfurreducens DL-1 cell culture and measurement were carried out under strict anaerobic conditions ( Fig. 2 ) with acetate and fumarate concentrations monitored over time. In short, 0.1 ml of early stationary phase cultures were injected into the measurement chamber at ~4 min (indicated by purple arrow in Fig. 3a ) after recording the stable baseline. To minimize the effect of external voltages and non-invasively probe the current output from individual cells, the short-circuit current was recorded at an acquisition rate of 10 Hz with a reference electrode/cathode (Ag/AgCl) grounded. Multiplex recordings on four electrodes from two separated wells, well 1 and well 2, exhibit independent, stepwise current increases after ~2 h ( Fig. 3a ). Each step consisted of two processes: an initiation by a fast-decaying peak, which might be attributed to the quick discharge of the cell membrane with accumulated electrons, followed by a stable plateau corresponding to sustained current output ( Fig. 3b ). Occurrences of these steps are not correlated between adjacent electrodes from the same well ( Fig. 3b ), indicating that (1) there is no cross-talk between electrodes and (2) the measured signals are localized to individual electrodes at the initial stage. Control experiment with dead DL-1 cells or acetate-depleted DL-1 cells did not yield detectable current ( Supplementary Fig. S1a,b ), which further demonstrates that the measured currents originate from cell metabolism versus interfacial impedance change. 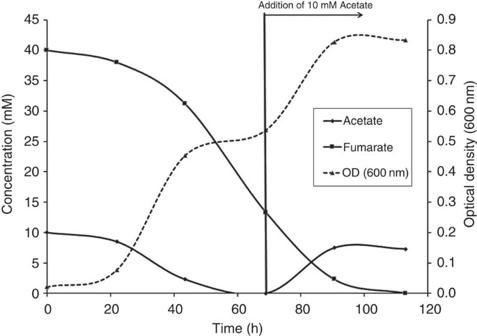Figure 2: Growth characteristics and carbon cycle forG. sulfurreducensDL-1. Growth of the inoculating culture was characterized using optical density at 600 nm with simultaneous measurement of acetate and fumarate concentration by HPLC. The growth phase was important to allow for reproducible results during replicate single-cell measurements. Cultures were utilized at early stationary phase, which was ~40 h after inoculation and 10 h before complete acetate consumption. Figure 2: Growth characteristics and carbon cycle for G. sulfurreducens DL-1. Growth of the inoculating culture was characterized using optical density at 600 nm with simultaneous measurement of acetate and fumarate concentration by HPLC. The growth phase was important to allow for reproducible results during replicate single-cell measurements. Cultures were utilized at early stationary phase, which was ~40 h after inoculation and 10 h before complete acetate consumption. 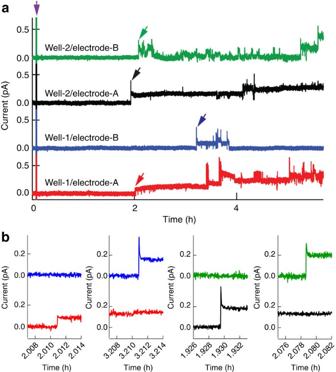Figure 3: Multiplex current recording at early stage of cell landing. (a) Short-circuit current recording on four selected electrodes that are characterized inFig. 1c. The purple arrow indicates the injection of DL-1 cells into the measurement chamber. The red, blue, black and green arrows mark the occurrence of the first current step on each electrode. (b) Zoomed view of the current steps marked ina. For comparison, the data from adjacent electrode in the same well are also plotted together. Full size image Figure 3: Multiplex current recording at early stage of cell landing. ( a ) Short-circuit current recording on four selected electrodes that are characterized in Fig. 1c . The purple arrow indicates the injection of DL-1 cells into the measurement chamber. The red, blue, black and green arrows mark the occurrence of the first current step on each electrode. ( b ) Zoomed view of the current steps marked in a . For comparison, the data from adjacent electrode in the same well are also plotted together. Full size image The amplitude distribution of the current steps recorded within the first 6.5 h features two peaks at 92 (±33) and 196 (±20) fA ( Fig. 4a , inset), which were consistent with single- and double-cell scenario, respectively. Further, phase-contrast microscopy was used during the experiment to monitor the cell position change around the measured electrode during electrical recording. When a DL-1 cell approached and physically made contact with the electrode surface, the short-circuit current increased to ~82 fA ( Fig. 4b ), indicating that the observed current was directly correlated with cell and electrode interaction. The contact of a two-bacterium assembly with measured electrode, correspondingly, leads to a larger current step of ~185 fA ( Fig. 4c ), showing that the current amplitude was determined by the number of cells that were involved in the interaction. Although every observed current step-up can be correlated with the cell–electrode interaction, it is worth mentioning that only ~30% of cell contact can translate into current output, which could be because of the requirement of optimal cell configuration for establishing electrical connection or the competition from residual fumarate as alternative electron acceptors. These results represent the first unambiguous characterization of the amount of current generated by a single Geobacter cell and also demonstrated direct electron transfer as the dominant electron pathway at DL-1/electrode interface outside a biofilm. 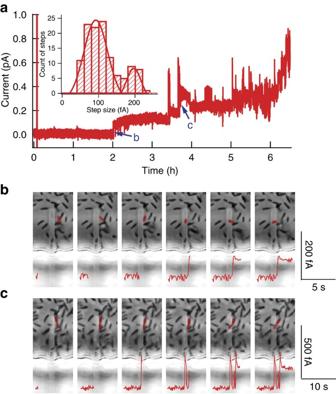Figure 4: Detailed analysis of the stepwise current output. (a) Short-circuit current data from electrode A from well 1 within the first 6.5 h. The arrows indicate the steps analysed inFig. 4b,c. Inset: statistic analysis of the amplitude distribution of the current steps inFig. 4a. (b,c) Evolution ofin situphase-contrast images of DL-1 cells on and around the measured electrode when a 82-fA (b) and 185-fA (c) step occurs, respectively. The current changes recorded at the same time are also included, and the cells that contact electrode concurrently with these current increases are marked in red. Figure 4: Detailed analysis of the stepwise current output. ( a ) Short-circuit current data from electrode A from well 1 within the first 6.5 h. The arrows indicate the steps analysed in Fig. 4b,c . Inset: statistic analysis of the amplitude distribution of the current steps in Fig. 4a . ( b , c ) Evolution of in situ phase-contrast images of DL-1 cells on and around the measured electrode when a 82-fA ( b ) and 185-fA ( c ) step occurs, respectively. The current changes recorded at the same time are also included, and the cells that contact electrode concurrently with these current increases are marked in red. Full size image Long-range charge transport studies The short circuit current was measured over time to probe how well the current output correlated with biofilm formation. As expected, as more cells landed into the well, the current steadily increased ( Fig. 5 ) while the measured open circuit voltage remained around 0.4 V versus Ag/AgCl. The generation of current and cell distribution around measured electrodes was first monitored and analyzed before the formation of a cell monolayer ( Fig. 5a ). Unlike the incremental current increases recorded within the first 6 h ( Fig. 5b , t1–t3), a dramatic rise of current output was observed for both electrodes in well 1 at almost the same time when the cell density approaches close packed ( Fig. 5b , t4). It is noteworthy that the cell number change on measured electrodes from t3 to t4 (~7–10 for electrode A and 6–8 for electrode B) were negligible compared with more than fivefold increase of current output. These results conclude that this dramatic current increase does not originate from direct cell–electrode interaction. Instead, these data indicate a more intimate cell–cell contact that triggers intercellular electron transfer through membrane proteins. As a result, cells remote from the measured electrode were also able to contribute to the current generation through long-range charge transport, leading to a higher current level consistent with literature precedents using biofilms [16] , [18] . 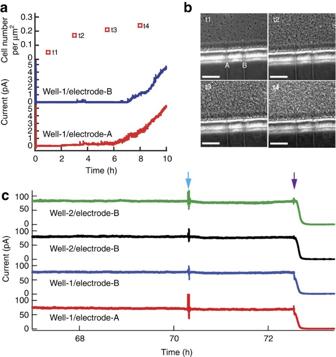Figure 5: Charge transport studies at longer time periods. (a) Short-circuit current recording from electrode A (red) and B (blue) in well 1 and correspondent monolayer cell density at 1 (t1), 3 (t2), 5.5 (t3) and 8 h (t4) after cell injection. (b) Phase-contrast optical images of cells around measured electrodes at t1–t4. Scale bars, 20 μm. (c) Short-circuit current recording at >60 h for electron transfer mechanism experiments. The cyan and purple arrows indicate flush by fresh media and biocide addition, respectively. Figure 5: Charge transport studies at longer time periods. ( a ) Short-circuit current recording from electrode A (red) and B (blue) in well 1 and correspondent monolayer cell density at 1 (t1), 3 (t2), 5.5 (t3) and 8 h (t4) after cell injection. ( b ) Phase-contrast optical images of cells around measured electrodes at t1–t4. Scale bars, 20 μm. ( c ) Short-circuit current recording at >60 h for electron transfer mechanism experiments. The cyan and purple arrows indicate flush by fresh media and biocide addition, respectively. Full size image Mechanism for electron transfer to electrodes Several experiments were performed to confirm whether the current generated by G. sulfureducens DL-1 was mediated by secreted soluble mediators in our system ( Fig. 5c ). First, the supernatant in the measurement chamber was carefully removed and replaced with fresh, N 2 /CO 2 (80/20) purged medium after 70 h. In contrast to the results from S. oneidensis MR-1 that showed >95% decrease in current amplitude after removing the soluble mediators [30] , the current retained >98% of original level in G. sulfurreducens DL-1, indicating that contributions from the mediated electron transfer process is negligible. Furthermore, after adding 0.1% glutaraldehyde as a biocide [32] to the measurement chamber, current generation was completely quenched within 30 min, verifying that the measured short-circuit current was associated with cellular metabolism rather than unknown electrochemical processes. We have further investigated the extracellular electron transfer using our first generation of nanoelectrodes in which an array of nanoholes (200 × 400 nm 2 ) precludes or single window (6 × 10 μm 2 ) allows for direct microbe/electrode contacts ( Supplementary Fig. S2 ) [30] . Despite the same exposed metal area between the two types of electrodes, current generation was only observed on the window electrode within the first 8 h, indicating the importance of Geobacter /electrode contact at the initial stage. This result is also in direct contrast with our previous measurement with S. oneidensis MR-1 cells, which gave almost identical current output between window and nanohole electrodes [30] . At longer times, it is interesting to note that the nanohole electrode was also able to yield a current, albeit at a much smaller magnitude, which could be attributed to the ability of G. sulfurreducens to grow electrically conductive pili or excrete proteins to overcome the nanohole barrier [23] , [24] , [25] . The complete mechanism of extracellular electron transport by EAB remains a matter of controversy and has raised growing discussion/debate in recent years [16] , [18] , [21] , [22] . In this work, we observed for the first time the quantized, stepwise current production in a model system, G. sulfurreducens DL-1. DL-1 current output was directly correlated with single-cell/electrode contact through in situ optical imaging. The amount of current generated per Geobacter cell is on the same order of magnitude as other estimates for Shewanella using time-dependent biofilm formation in a MFC (80–200 fA per cell) [33] or Shewanella precultured at +200 mV versus Ag/AgCl (200 fA per cell) [31] . The results from DL-1 differ significantly from our previous studies involving S. oneidensis MR-1 because of the presence of soluble redox mediators, which allowed for current generation independent of cell and electrode contact [30] . Combined with experiments designed for studying electron transfer mechanisms after biofilm formation, these results unambiguously demonstrate that direct electron transfer was the dominant mechanism used by DL-1 cells. However, the use of the wild-type strain does not allow for the impact of residual exopolysaccharide matrix associated with single cells to be ascertained. The results from these single-cell measurements also represents a unique insight into electron transfer from Geobacter . Biofilms (of various thickness) are typically formed on interdigitated electrodes and the long induction times to observe current from these systems has led researchers to conclude that electrode attachment is required for the expression of extracellular electron transfer proteins [26] , [27] . However, our results suggest an entirely different mechanism where immediate attachment of Geobacter leads to a stepwise current increase and that developed biofilm studies are observing electron transfer mediated by bulk biofilm conductivity in addition to the impact of quorum sensing. Time-dependent gene transcription biofilm studies of early-stage Geobacter biofilms on conductive and non-conductive supports would provide valuable data for this argument but is currently outside the scope of this work. The single-cell study of current generation and charge transport also enabled the estimation of the intrinsic limit of MFC current density, which could be simplified by dividing the single DL-1 current output with cell volume. This gave a value of ~10 6 A m −3 , which was 2–3 orders of magnitude higher than the best volumetric current density reported in working MFCs [34] , [35] , [36] , and more than one order of magnitude higher than the value obtained from G. sulfurreducens DL-1 biofilm studies [37] . The current experiments do not address potential stratification related to electron transfer as thicker biofilms are formed (>400 μm) but does present a compelling support for the theory that individual cells outside a biofilm are unilaterally active, whereas their inclusion in biofilms results in potential deactivation to sustain the bacteria in the biofilm [38] . Although this estimation was very crude and could only serve as the upper bound limit, it does suggest that the low current density of state-of-the-art MFCs is not limited by the current generation capability of EAB, and there is substantial room for improvement through novel electrode architectures. Growth of G. sulfurreducens DL-1 DL-1 was grown from frozen 50% dimethyl sulfoxide stocks (generated from cultures provided by D. Lovley, UMass Amherst) in sterile sealed tubes containing 10 ml of freshwater media degassed with a N 2 /CO 2 (80/20) gas mixture [22] , [39] . All transfers were performed in the 80/20 gas mix. Approximately 30 min ahead of inoculating the media with Geobacter , 0.1 ml of a sealed L -cysteine solution (0.1 M) degassed with nitrogen and sterilized via autoclave (15 min, 121 °C) was added to the media under the gas mix atmosphere. This step was essential as it was the partially decomposed cysteine used in this step that eliminated residual oxygen from the culture media. This reduced form of cysteine also reacted with the fumarate as observed from the shift of the fumarate peak during HPLC analysis (data not shown). Without this preparation of cysteine, inoculation with the frozen stocks did not result in cellular growth. Cysteine was not detected after the 30 min by HPLC. Cells were grown with 10 mM acetate at 30 °C. The first subculture after 48 h of growth from the frozen stock was used for growth experiments as well as with inoculating the measurement chamber. No current was observed when cells were not present in the electrode system. Aliquots were removed periodically during each growth experiment for analysis by HPLC (Varian, Inc.) with a refractive index detector. The mobile phase was a 5-mM sulphuric acid solution and the column was PL Hi-Plex H + ion exchange column (60 °C) at a flow rate of 0.6 ml min −1 . Variable concentration standards of acetate, lactate and fumarate were calibrated using the HPLC method and for peak identification. The aliquots were centrifuged (3 min, 20,000 g , 22 °C) to pellet the bacteria and insoluble particles. Following centrifugation, sample supernatants were syringe filtered with a 0.2-μm polytetrafluoroethylene (Fisher Scientific) filter and stored at 4 °C before analysis by HPLC. Freshwater medium formulation In 1 l of 18 MΩ water, the following components were mixed: 30 mM of sodium bicarbonate, 4.7 mM of ammonium chloride, 3.8 mM of sodium potassium monobasic and 1.3 mM of potassium chloride. In addition, 10 ml of both a stock vitamin solution [40] and mineral solution [41] were incorporated. Sodium acetate (10 mM) and 40 mM of sodium fumarate were added as carbon sources. After proper mixing, the appropriate aliquots were gassed with 20.06% carbon dioxide-balanced nitrogen mix (Airgas, Inc custom gas mixture) and anaerobically sealed, before autoclaving at 121 °C for 15 min. Cell cultures for nanoelectrode measurements Before inoculation of the measurement chamber, the culture media were contained in anaerobic pressure tubes with butyl rubber stoppers under an 80% N 2 -20% CO 2 atmosphere and grown at 30 °C for 48 h with ~10–15 mM fumarate remaining in the culture medium. Optical density at 600 nm of the inoculating cultures was 0.3–0.4 before adding 0.1 ml of the culture to the measurement chamber. The measurement chamber contained degassed 10 mM acetate in 0.9 ml freshwater medium. Chip fabrication Glass substrates (50 × 22 mm 2 , 0.17 mm thick; VWR) were cleaned in Piranha solution (3:1 concentrated sulphuric acid to 30% hydrogen peroxide) for 30 min, rinsed with deionized water (15 s), acetone (15 s), isopropanol (15 s) and dried in N 2 flow. A two-layer photoresist consisting of LOR3A and S1805 (Microchem) was sequentially deposited by spin coating, and baked for 5 min at 185 °C and 115 °C, respectively. The metal electrodes were defined by photolithography, followed by thermal evaporation of 2 nm Ti and 8 nm Au. Each glass chip has 32 finger electrodes (2 μm wide) defined at the chip centre with fan out wiring to I/O points at the two ends of the chip. The finger electrodes were arranged in 16 groups of two parallel electrodes that are 20 μm apart, and the distance between adjacent groups is 250 μm. After lift-off, a ~40-μm thick SU-8 layer was uniformly deposited and pre-baked at 95 °C for 30 min. Photolithography was then used to define different-sized wells around the finger electrode tips. The positions of wells were precisely controlled so that all electrodes exposed the same metal area of 24 μm 2 . After post-baking at 60 °C for 2 h and development, the chip was hard-baked at 180 °C for 30 min. Finally, organic residues were removed from the electrodes by ultraviolet ozone treatment for 2 min at 200 °C. Electrochemical measurements All measurements were carried out in a two-electrode configuration because of the small current levels [42] , [43] , with Ag/AgCl as both cathode and reference electrode. The millimeter-scale Ag/AgCl electrode has 5–6 orders of magnitude larger surface area than the anodes (microelectrodes); hence this would not be the limiting factor even in long-term experiments. The current at the working electrode was detected using a current preamplifier (1211; DL Instruments, Inc.) with a gain of 10 9 –10 11 V/A. The amplified signals were digitized using a multichannel analogue-to-digital converter (Digidata 1440A; Molecular Devices). The Digidata 1440A was also used to apply potentials during cyclic voltammetry measurements, with a typical sweep rate of 10 mV s −1 . The whole electrochemical cell was housed in a Faraday cage, yielding a noise level of <40 fA. All experiments were performed with more than 20 independent measurements across five different devices. Cell measurements and in situ optical imaging The short-circuit current was recorded at an acquisition rate of 10 Hz with reference/cathode electrode grounded. A polydimethylsiloxane housing was incorporated to the outside of the inner measurement chamber, allowing for continuous or batch solution exchange, and control of anaerobic atmosphere by continuously flowing 20 sccm N 2 /CO 2 (80/20) gas mixture during measurement ( Supplementary Fig. S3 ). In situ optical imaging was carried out with an inverted phase-contrast microscope (IX71; Olympus Inc.) and × 100 oil-immersion lens. A 518.5–699.5-nm bandpass filter (FF01-609/181; Semrock) was applied after the lamp house to block ultraviolet and infrared light that are known to be hazardous to cells in long-term recording. Flush and biocide control experiments For the flush experiment, the supernatant in the measurement chamber was carefully removed with a syringe, and then 1 ml N 2 /CO 2 (80/20) purged media was added to the chamber. The process was repeated twice to insure removal of all possible mediators in the measurement chamber. For the biocide experiment, 0.1 ml 1% glutaraldehyde was injected into the measurement chamber (containing ~1 ml solution), leading to final glutaraldehyde concentration of ~0.1% with minimal dilution of other species. Estimation of single- Geobacter current density In this calculation, the space of other components of the MFC (anode, cathode, electrolyte and so on) were ignored and only the volume of a single bacterial cell was considered, which was ~10 −19 m 3 based on a cylindrical model with 300-nm diameter and 1.5-μm height. The current output per Geobacter cell, according to Fig. 4a , was 92(±33) fA. As a result, the intrinsic limit of current density for Geobacter DL-1 cells was estimated to be on the order of 10 6 A m −3 . Similarly, the volumetric current density in G. sulfurreducens DL-1 biofilm studies [37] was approximated by dividing the projected area-based current density (3.5 A m −2 ) with biofilm thickness (50 μm), which gives the value of 7 × 10 4 A m −3 . How to cite this article: Jiang, X. et al. Probing single- to multi-cell level charge transport in Geobacter sulfurreducens DL-1. Nat. Commun. 4:2751 doi: 10.1038/ncomms3751 (2013).